Nothosaur foraging tracks from the Middle Triassic of southwestern China The seas of the Mesozoic (266–66 Myr ago) were remarkable for predatory marine reptiles, but their modes of locomotion have been debated. One problem has been the absence of tracks, although there is no reason to expect that swimmers would produce tracks. We report here seabed tracks made by Mesozoic marine reptiles, produced by the paddles of nothosaurs (Reptilia, Sauropterygia) in the Middle Triassic of the Luoping localities in Yunnan, southwestern China. These show that the track-making nothosaurs used their forelimbs for propulsion, they generally rowed (both forelimbs operating in unison rather than alternately), and the forelimb entered medially, dug in as the paddle tip gained purchase, and withdrew cleanly. These inferences may provide evidence for swimming modes, or it could be argued that the locomotory modes indicated by the tracks were restricted to such contact propulsion. Such punting behaviour may have been used to flush prey from the bottom muds. The seas of the Mesozoic differed from those before and after in that top predators were reptiles, primarily diapsid reptiles. Mesozoic marine reptiles included, at times, sauropterygians, ichthyosaurs, crocodilians, turtles, mosasaurs, and several minor clades. Most of these are thought to have used powerful lateral movements of their tails and posterior regions of the trunk in propulsion, whereas the sauropterygians variously rowed, paddled or ‘flew’ through the water, mainly using their forelimbs to generate forward propulsion [1] , [2] , [3] , [4] , [5] . Understanding the locomotion of these diverse animals, generally the top predators in their communities, and adopting a broad range of carnivorous diets, is important in comprehending Mesozoic marine ecosystems. Marine reptiles radiated dramatically in Early and Middle Triassic seas following the devastating Permo-Triassic mass extinction. That event had killed as many as 90–95% of all species on land and in the sea, and the recovery of life was delayed for 5–10 million years (Myr) by a combination of biological causes, primarily the profundity of the extinction and destruction of key life modes such as forests on land and reefs in the sea, as well as physical environmental causes, primarily repeated global warming crises in the Early Triassic [6] , [7] . The first marine reptiles—ichthyosaurs, hupehsuchids, nothosaurs and pachypleurosaurs—are known from the late Early Triassic, for example the Chaohu assemblage of southeastern China [8] , and further new clades, including placodonts, and possibly thalattosaurs emerged soon after, in the early Middle Triassic. These marine reptiles swam in shallow seas worldwide, feeding generally on small to large prey ranging from crustaceans and other invertebrates to fishes. In addition, the larger marine reptiles, such as some ichthyosaurs, thalattosaurs and nothosaurs, may also have fed on smaller marine reptiles, while the placodonts specialized in browsing and crushing oysters. Following the end-Triassic mass extinction 201 Myr ago, ichthyosaurs and plesiosaurs diversified in the Early Jurassic and these clades, and later mosasaurs, were important predators in marine ecosystems throughout the Jurassic and Cretaceous. For all this substantial predatory activity by a broad diversity of marine reptiles throughout the 187 Myr of the Mesozoic, reports of tracks or markings made by sauropterygians or ichthyosaurs are rare [9] , [10] , and not very convincing. This is surprising, as fishes and tetrapods today commonly make markings on the seabed when they are foraging or moving, and indeed some rare examples of sinusoid impressions produced by the ventral fins of fishes have been reported (for example, refs 11 , 12 ). Here we report a large surface from the Guanling Formation, near Daaozi Village, Luoping, Yunnan Province, China ( Fig. 1a ), covered with 350 regular impressions that are interpreted as paddle prints made by a nothosaur, or nothosaurs, as they propelled themselves across the seabed. This new discovery confirms some previous assumptions about the modes of locomotion and feeding by these early sauropterygians, and suggests some other, unexpected behaviours, such as foraging on startled prey in clouds of disturbed seabed mud. 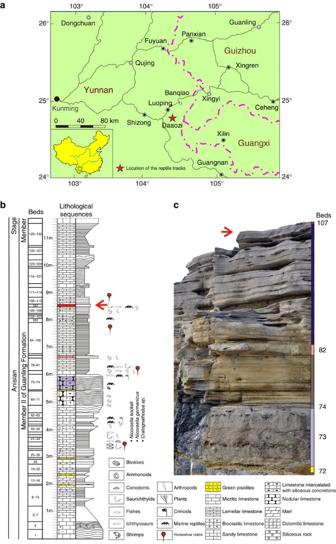Figure 1: Location and stratigraphic horizon of the Luoping marine reptile paddle prints. (a) Location map of Yunnan and Guizhou provinces, southwestern China, showing the Luoping (Daaozi village) location. (b) Sedimentary log through the Guanling Formation at the Daaozi locality, showing lithologies, sedimentary structures and key fossiliferous beds, including the footprint layer (top of bed 107). The conodontsNicoraella germanicus, N. kockeli, andCratognathodussp. occur only in beds 41 and 43. (c) Photograph of beds 72–107, immediately below the footprint horizon, which is marked by an arrow. Figure 1: Location and stratigraphic horizon of the Luoping marine reptile paddle prints. ( a ) Location map of Yunnan and Guizhou provinces, southwestern China, showing the Luoping (Daaozi village) location. ( b ) Sedimentary log through the Guanling Formation at the Daaozi locality, showing lithologies, sedimentary structures and key fossiliferous beds, including the footprint layer (top of bed 107). The conodonts Nicoraella germanicus, N. kockeli , and Cratognathodus sp. occur only in beds 41 and 43. ( c ) Photograph of beds 72–107, immediately below the footprint horizon, which is marked by an arrow. Full size image Discovery The tracks were first discovered on top of bed 43 (associated with protorosaur skeletal fossils) and beds 32 and 34, in April 2009 during the first fossil excavation in quarry 1 of the Luoping biota, exposing the Shangshikan section [13] . Much more abundant and varied trace fossils were then found during the second excavation, in quarry 2 (Menqianpo section). These tracks occur on bed 107 ( Fig. 1b ), higher in the section than the isolated finds from the Shangshikan section. The track-bearing surface, comprising micrite and marls, was excavated and cleaned by teams of students and farmers ( Supplementary Fig. 1 ), and this is described in detail here. The other track-bearing layers showed only isolated specimens, and these are not reported further here. These sites are part of the Luoping National Geopark, established in 2011 in recognition of the unique fossils and their quality. Sedimentology and stratigraphy The track finds occur at different levels (beds 32, 34, 107) in Member II of the Guanling Formation [8] , [13] . The Guanling Formation occurs extensively throughout eastern Yunnan and western Guizhou provinces, following conformably above the Jialingjiang Formation, and succeeded by the Yangliujing Formation [8] , [13] . It is dated as Anisian, spanning the Aegean, Bithynian, Pelsonian and lower Illyrian substages, based on evidence from conodonts and radiometric dating. When fully developed, the Guanling Formation is over 900 m thick, and Member II is 580 m thick, comprising a succession of dark nodular micritic limestone, muddy limestone and cherty micritic limestone with bands of dolomite. The tracks and the Luoping biota occur only in the upper part of the Guanling Formation (Member II), and this is dated by abundant conodonts that are assigned to the Nicoraella kockeli Zone [14] , characteristic of the Pelsonian Substage of the Middle Triassic Anisian Stage [15] . The Luoping biota The fossil tracks are associated with the Luoping biota [13] , [14] , [16] , which occurs in the middle part of Member II of the Guanling Formation. Near the village of Daaozi (Dawazi), the Shangshikan section, a 16-m-thick succession of richly fossiliferous beds, is exposed, delimited at the bottom by bioturbated limestone and at the top by silty limestone ( Fig. 1b, c ). The fossiliferous horizons comprise mainly thinly laminated micritic limestone alternating with thin- to moderately thick-bedded silty limestone. Lower units (Beds 2–66) are dark grey, medium- to thick-bedded, laminated micritic limestones with siliceous concretions. Grey–yellow, thin-bedded silty mudstones (Beds 14, 17, 24 and 72) are pronounced in the lower units. A highly diverse fish assemblage has been recovered mainly from Beds 33 and 44. Most of the saurichthyid fish fossils are found in Bed 48. Beds 57 and 61 yield marine reptiles, associated with shrimps, crinoids and plant fossils. These units are followed by a 1.4-m-thick succession of dark grey medium- to thick-bedded nodular limestone intercalated with cherty concretions (Beds 67–74). The overlying 2.9 m of dark grey to yellowish–grey laminated muddy limestone (Beds 75–110) contains rare siliceous concretions. Numerous marine reptiles along with rare shrimps occur in Beds 78–81 and 106. These highly fossiliferous units within a restricted rock sequence comprise the Luoping biota [13] , [14] , [16] . So far, nearly 20,000 individual macrofossils have been collected at Daaozi in several closely located quarries. Arthropods dominate by far, comprising over 90% of the fauna, followed by fishes (4%), then bivalves (2%), and then relatively tiny proportions (<1%) of plants, gastropods, marine reptiles and others [13] . The dominant arthropods include remarkable materials of crustaceans, millipedes and horseshoe crabs. The majority are crustaceans, including decapods (lobsters and shrimps), isopods, cycloids, mysidiaceans, conchostracans and ostracods. These arthropods fed on plankton-sized prey and plants, and were in turn preyed on by bony fishes, which formed food for predatory fishes such as Saurichthys as well as small, medium and large marine reptiles [13] . The track surface The tracks are preserved on a single bedding plane, on top of bed 107 ( Fig. 1 ), measuring maximally 22 m by 10 m in exposed area, with a total of 125 m 2 photographed and recorded ( Fig. 2a , Supplementary Figs 2–4 ). The surface is gently undulating, with a generally smooth surface, indicating gentle conditions of deposition, and the existence of a cohesive, partially solidified seabed at the time of track formation. Here and there, small trails and paired impressions ( Isopodichnus ) formed by worms and crustaceans are evident. There are occasional longer impressions, slightly undulating and some 10 mm wide and up to 1 m long, probably gastropod or worm trails, but conceivably tail markings by marine reptiles; these, however, are not apparently associated with any paddle trails. Several fish specimens occur on the surface, identified as the chondrosteans Saurichthys and Sinosaurichthys, the ‘sub-holostean’ Placopleurus and the holostean Sangiorgioichthys , as well as small crustaceans, gastropods, bivalves and plants. These details have been little modified by modern erosion because most of the site represents a freshly cleared surface, exposed by splitting and lifting the overlying slabs, so the exact relationship of prints and overlying moulds could be seen ( Supplementary Fig. 5 ). 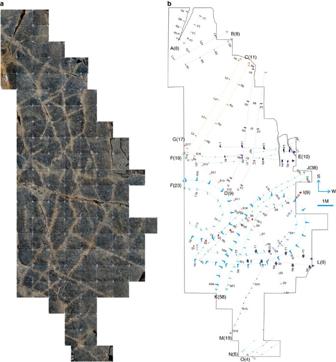Figure 2: Overview of the footprints and the main trackways. The trackways are distinguished as series A–O. (a) Photographic plan, made from a composite of 124 images, each of a 1-m2light-coloured lines are cracks in the rock surface. (b) Sketch plan of the site, showing all tracks. Arrows indicate direction of movement in each case. Figure 2: Overview of the footprints and the main trackways. The trackways are distinguished as series A–O. ( a ) Photographic plan, made from a composite of 124 images, each of a 1-m 2 light-coloured lines are cracks in the rock surface. ( b ) Sketch plan of the site, showing all tracks. Arrows indicate direction of movement in each case. Full size image There are 350 individual paddle markings, with 247 of these organized into 15 trackways, each comprising multiple imprints (4–58 prints per trackway, mean=16.5; Supplementary Tables 1 and 2 ). Twelve of the imprints are paired, with left and right-hand prints forming mirror images of each other, whereas three trackways (labelled G, I and M) are single series of prints. Of the paired trackways, their 202 prints mainly comprise matching pairs, but there are some unpaired prints at the ends of rows, where the trackway disappears under an overlying stratum or off the edge of the cliff. Track and print dimensions The term ‘track’ as commonly used may be ambiguous, sometimes referring to a single imprint made by the impression of a single limb, and at other times to a series of such imprints. In the descriptions, we distinguish individual imprints or prints from trackways of multiple prints. We use the term ‘pace’ to refer to the distance between successive imprints made by the same limb as the animal moved forward. We use the term ‘track’ only in broadly descriptive portions of the paper, when it refers in a general sense to the individual imprints and the trackways as a whole. The trackways show considerable variation in width (distance between the outer tips of the left and right series of prints), ranging from 35 to 67 cm ( Table 1 ). Trackway widths do not show continuous variation, but divide into two clusters, presumably indicating animals of different body sizes, namely small (35–42 cm) and large (50–67 cm) clusters ( Fig. 3a ). The ‘large’ category could be further divided perhaps into medium (50–52 cm) and large (56–67 cm) imprints ( Fig. 3a ), but this subdivision may simply reflect the small sample size and the broad range of dimensions in the larger prints, as suggested by the comparison of trackway and print widths ( Fig. 3c ). The size classes broadly match the range of mean pace lengths ( Table 1 , Fig. 3b ), but not exactly. This is because animals may adopt differing pace lengths depending on their speed of movement over the seabed. So, for example, trackway F, with an overall width of 36 cm shows a mean pace length of 78.9 cm, whereas trackway J, with a similar width of 38 cm shows a mean pace length of 45.6 cm, suggesting that its producer was moving in a rather more languid fashion. Table 1 Summary of key measurements of the 15 trackways from the Guanling Formation in southwestern China. 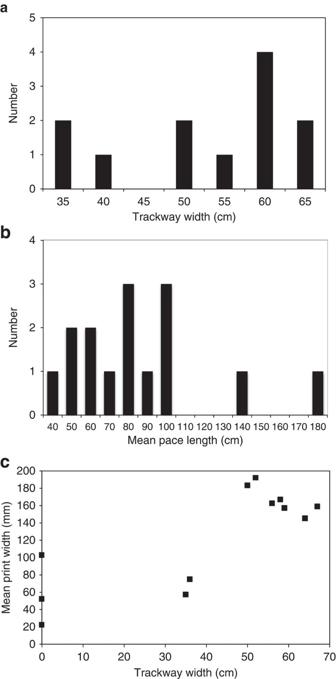Figure 3: Dimensions of the 15 individual trackways. (a) Number of trackways of different mean widths. (b) Number of trackways showing different mean pace lengths. (c) Plot of mean paddle widths and trackway widths. Full size table Figure 3: Dimensions of the 15 individual trackways. ( a ) Number of trackways of different mean widths. ( b ) Number of trackways showing different mean pace lengths. ( c ) Plot of mean paddle widths and trackway widths. Full size image Individual prints are broad, measuring 4.1–19.6 cm from side to side (medio-laterally), and showing variable antero-posterior dimensions. The medio-lateral measurements are recorded ( Fig. 3c ; Supplementary Table 3 ), but the antero-posterior dimension is less informative because it depends on a combination of the body size of the animal and the behaviour: individual prints can vary from narrow slots in the sediment to longer imprints made by the paddle dipping and sweeping back. Mean print width is proportional to overall trackway width (Pearson product moment correlation coefficient, 0.725, P =0.027), and there appear to be two size categories ( Fig. 3c ), small (print width 55–80 mm; trackway width 35–42 mm) and large (print width 140–200 mm, trackway width 50–67 cm). The three points with zero trackway width ( Fig. 3c ) are the three single-sided trackways (G, I and M). Systematics The trace fossils described here are unique in morphology, and so are established as a new ichnotaxon. Dikoposichnus ichnogen. nov. Type ichnospecies Dikoposichnus luopingensis ichnosp. nov. Meaning of names The genus name is based on ancientGreek (dikopos), meaning two-oared, a term generally applied to ships rather than marine reptiles. The species name honours the locality and the Luoping biota. Type specimen Trackway E, Menqianpo, near Daaozi village, Luoping, Yunnan Province, China ( Figs 2 and 4g,h , Supplementary Figs 2 –4 and 10). Casts and Lidar scan data of this trackway, and of all tracks from the whole site, as described here, are retained in the Chengdu Center of China Geological Survey. 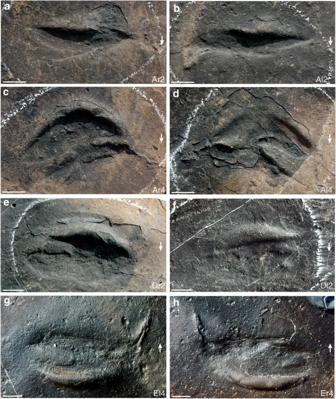Figure 4: Examples of individual paddle prints. (a) Sigmoid print Ar2. (b) Sigmoid print Al2. (c) Double-hit print Ar4. (d) Double-hit print Al4. (e) Double-hit print Dr2. (f) Double-hit print Dl2. (g) Sigmoid print with a point laterally El4. (h) Sigmoid print with a point laterally Er4. The three-character notation for each imprint indicates the trackway designation (A–O), whether the print is from left (l) or right (r), and the number of the imprint. Direction of movement is shown by arrows. Scale bar, 3 cm. Figure 4: Examples of individual paddle prints. ( a ) Sigmoid print Ar2. ( b ) Sigmoid print Al2. ( c ) Double-hit print Ar4. ( d ) Double-hit print Al4. ( e ) Double-hit print Dr2. ( f ) Double-hit print Dl2. ( g ) Sigmoid print with a point laterally El4. ( h ) Sigmoid print with a point laterally Er4. The three-character notation for each imprint indicates the trackway designation (A–O), whether the print is from left (l) or right (r), and the number of the imprint. Direction of movement is shown by arrows. Scale bar, 3 cm. Full size image Diagnosis Double row of imprints, preserved as concave epireliefs (bed) or convex hyporeliefs (sole). Each imprint is a narrow V-shaped, slot-like depression, with a mound of sediment behind. Individual imprints may be elliptical to sigmoid-shaped in plan view, sometimes with an anterior sweep at the medial edge. Individual imprints are transverse to the direction of travel, spaced widely apart and with variable pace length. When preserved as trackways, prints generally occur in matching pairs, suggesting the limbs moved in concert, but they may be offset, produced by alternate left-right pacing. Overall trackway width is 30–70 cm, and individual prints are 5–20 cm along their longest axis, transverse to the direction of movement. Occasionally comprises a single trackway of prints. Variation in paddle print morphology The different trackways show considerable variation in the form of the individual paddle imprints, and these are interpreted as a result of variations in the mode of locomotion and the precise interaction of the paddle and the sediment. Typical prints ( Fig. 4a,b,g,h ) show a slightly sigmoid, curved shape in plan view, with a point laterally, and a forwards and inwards sweep medially. The bottom of the impression runs from shallow medially to much deeper at mid-print, and slightly shallower laterally. Left and right-hand prints form mirror images of each other. There is a substantial mound of sediment behind the mid portion of the imprint, and this mound can be used to interpret the direction of movement of the producer, lying as it must behind the print, as the animal dug in its paddle tip and pushed backwards to propel the body forward. These print types are seen in trackways A and E ( Supplementary Figs 6,10 and 16 ). The leaf-like impression and semicircular imprints may have been produced by a slight or a strong scull, respectively ( Supplementary Fig. 6d–g ). A second print type is more elliptical in shape, and lacks the medial sigmoid curve ( Figs 5b,c and 6e,f ). These prints are as deep as the first type, but the posterior sediment mound has a straight anterior margin and a curved posterior margin. Importantly, the limbs were moving with alternate left and right pacing in these cases. This print type is seen in trackways B, F and J ( Supplementary Figs 7 and 13 ). 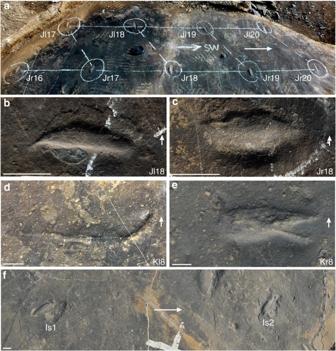Figure 5: Examples of individual paddle prints. (a) Four pairs of prints of Type J. (b) Elliptical Jl18. (c) Elliptical Jr18. (d) Leaf-like Kl8. (e) L-shaped Kr8. (f) Two single prints of single Type I. The three-character notation for each imprint indicates the trackway designation (A–O), whether the print is from left (l) or right (r), and the number of the imprint. Direction of movement is shown by arrows. Scale bar, 3 cm. Figure 5: Examples of individual paddle prints. ( a ) Four pairs of prints of Type J. ( b ) Elliptical Jl18. ( c ) Elliptical Jr18. ( d ) Leaf-like Kl8. ( e ) L-shaped Kr8. ( f ) Two single prints of single Type I. The three-character notation for each imprint indicates the trackway designation (A–O), whether the print is from left (l) or right (r), and the number of the imprint. Direction of movement is shown by arrows. Scale bar, 3 cm. 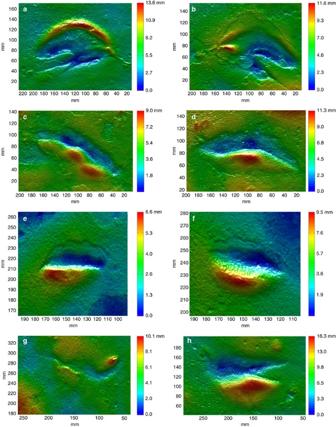Figure 6: Examples of individual paddle prints. (a) Double-hit print Ar4. (b) Double-hit print Al4. (c) Sigmoid print El2. (d) Sigmoid print Er3. (e) Elliptical Jl18. (f) Elliptical Jr18. (g) Leaf-like Kl8. (h) L-shaped Kr8. These are two-dimensional images of 3D models, colour-coded to indicate relief. Direction of movement is indicated by the sediment mound,behindeach print (shown by red highlight). Scale is indicated by centimetre divisions along the sides of each image. Full size image Figure 6: Examples of individual paddle prints. ( a ) Double-hit print Ar4. ( b ) Double-hit print Al4. ( c ) Sigmoid print El2. ( d ) Sigmoid print Er3. ( e ) Elliptical Jl18. ( f ) Elliptical Jr18. ( g ) Leaf-like Kl8. ( h ) L-shaped Kr8. These are two-dimensional images of 3D models, colour-coded to indicate relief. Direction of movement is indicated by the sediment mound, behind each print (shown by red highlight). Scale is indicated by centimetre divisions along the sides of each image. Full size image A number of the imprints show double impressions. The first of these is elliptical and shows two mounds behind the print, set at a slightly oblique angle, seen in trackways C and D ( Supplementary Figs 8,9 and 16d,g,h ). There is a larger medial mound, with a smaller lateral mound partly in front. The second kind of double impression, as seen in trackway L ( Supplementary Figs 15 and 16e,f ), is paired and branched, and is also seen in bed 32, 34 and 43 of quarry 1. The limb movements are alternate rather than synchronous. The third kind of double-hit imprint is seen in trackways H and K ( Supplementary Fig. 14 ), and is paired, asymmetrical, and has a leaf-like left-hand print and an L-shaped right-hand print. Markings in the single trackways (G, I, M) are similar to those in the double trackways. In trackway G ( Supplementary Figs 11a,b,c and 16b ), the imprints are elliptical and show a small mound anteriorly and posteriorly. In single trackway I ( Supplementary Figs 14 and 16a ), individual prints are 14-cm wide, and really just low sediment mounds, elliptical in outline, with one sharp edge indicating the back of the print, but only a minimal hollow impressed in the sediment and with a low posterior mound. In single trackway M ( Supplementary Fig. 11d–g ), prints are shallow elliptical pits, 5-cm wide on the transverse axis. Mode of track formation The individual imprints and the morphology of the complete trackways suggest that they were formed by a limbed animal moving in a steady manner over the seabed. Individual imprints suggest a mode of formation in which the paddle touched bottom first close to the midline (medially), swept round and entered the sediment to a depth of several centimetres, pushed backwards raising the sediment mound, and exited from the sediment, leaving a lateral point ( Fig. 7 ). 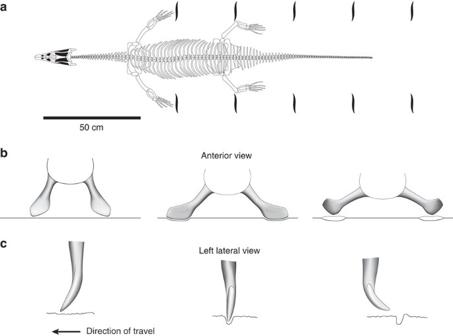Figure 7: TheDikoposichnustrack and its likely maker. (a) Skeleton ofLariosaurus, viewed from above, paddling along and producing the tracks with its front paddles. (b,c) Possible paddle movements as the nothosaur swims forward, leaving the trackway, shown in anterior (b) and lateral (c) views. Figure 7: The Dikoposichnus track and its likely maker. ( a ) Skeleton of Lariosaurus , viewed from above, paddling along and producing the tracks with its front paddles. ( b , c ) Possible paddle movements as the nothosaur swims forward, leaving the trackway, shown in anterior ( b ) and lateral ( c ) views. Full size image Most of the trackways show synchronous movements in which the forelimbs touched bottom at the same time, and presumably pushed back together. Four trackways, B, F, J and L, however, show alternate pacing, with left and right-hand prints impressed at mid-pace length of the other side. The synchronous and alternate limb motions could presumably have been produced by the same species of animal, in that most modern tetrapods can adopt either gait depending on speed ( cf . the trot and gallop of a horse). Here we see no relation between gait and trackway size, so it is likely animals of any size could produce either motion style. Further, it is probably meaningless to attempt to calculate speed of movement: the standard techniques used with terrestrial trackways depend on a constant relation between speed and pace length, but here pace length can vary according to whether the animal touches down or not, and how much it floats forward between punts. Some imprints show double patterns of different kinds ( Supplementary Figs 9 and 14 ). The first example, with double posterior mounds ( Supplementary Fig. 9 ) could suggest perhaps a backwards shove by the paddle, followed by a second dip into the sediment and a second push at the lateral end of the paddle ( Fig. 6g,h ). This type might have been interpreted as a combined imprint produced first by the fore-paddle and then by the hind-paddle of the same side, but it is unlikely that the hind-paddle could dip so precisely into the print already formed by the fore-paddle, and without deepening or otherwise affecting the grooved portion. The double imprints seen in trackway L, on the other hand ( Supplementary Figs 15 and 16e,f ), show double markings of the paddle rather than simply double mounds. The doubling is especially clear laterally, and it cannot be said for sure whether these represent double hits by the fore-paddle or imprints by fore- and hind-paddle in succession. The former interpretation is more likely for two reasons: (1) the medial insertion of the propulsive organ is identical in each case, with no evidence that the second imprint was not directly overprinted on the existing groove, and (2) likely track makers such as nothosaurs (see below) have hindlimbs that were generally shorter than the forelimbs, and would likely have produced imprints in a separate series medially of the forelimb markings ( cf. Fig. 7 ). In the single-line trackways G, I and M ( Supplementary Figs 11,12 and 16a,b ), it is hard to determine whether the matching series of imprints has not been found, or the animal was paddling with one foot. All single-line trackways, however, are straight and not curving, so the animal was evidently not cornering, but using a single paddle to propel itself in a single direction. Perhaps these animals were swimming across a bottom current, and such a single-dipping mode, with the other paddle working against the water, would ensure a straight, rather than downstream, direction of travel. Identity of the track maker In identifying the track maker, the obvious culprits are marine reptiles; the size of the tracks rules out arthropods or fishes. It is likely that the imprints were made by the forelimbs, for two reasons: (a) there is no case of a print of a putative hindlimb or foot overprinting a forelimb print, and (b) Mesozoic marine reptiles generally used their forelimbs much more actively than their hindlimbs in locomotion [1] , [2] , [3] , [4] , [5] . There appear to have been two size classes of track makers at Luoping, based on estimated torso width. Torso width can be estimated by measuring the inner width of the trackways (spacing between medial edges of paired imprints), and adding an additional distance on each side for the length of the humerus. Note that the maximum trackway width is probably less than the total width of the track maker with forelimbs extended, because the forelimbs would have been bent down and inward to the sides of the torso to push against the seabed. Thus, the outer trackway widths of small (35–42 cm) and large (50–67 cm) sizes ( Fig. 3b ) point to animals with torsos about 25–30 cm and 30–45 cm wide, allowing for the 5–10 cm wide paddle imprints on each side. The marine reptiles from Luoping, and the slightly younger Panxian locality, include ichthyosaurs, nothosaurs, pachypleurosaurs, placodonts, protorosaurs and saurosphargids ( Supplementary Table 1 ). The pachypleurosaurs can be ruled out as too small (length 10–20 cm). The protorosaur, the placodont and the saurosphargids have distinct fingers with long claws, and yet there are no traces of individual finger or claw marks in the 247 Luoping tracks. Further, placodonts and saurosphargids generally have short hands, and protorosaurs have long-fingered lizard-like hands, and it is not clear how, for any of these groups, their hands could have been bent sideways to produce the prints reported here. For these two reasons, these three groups are ruled out as potential track makers. Of the remaining marine reptiles, the ichthyosaurs powered their swimming by lateral whole-body or tail sweeps [17] , so it is unlikely they would have deployed their paddles in pushing locomotion. Further, although ichthyosaur paddles extended beneath the belly in life, these were single stiff structures that could only have produced fan-like sweeping marks as they moved from a fully extended lateral position to a backwards-oriented, parasagittal position, at right angles to the starting point. This leaves the nothosaurs Lariosaurus and Nothosaurus as the most likely track makers ( Figs 7a and 8 ). 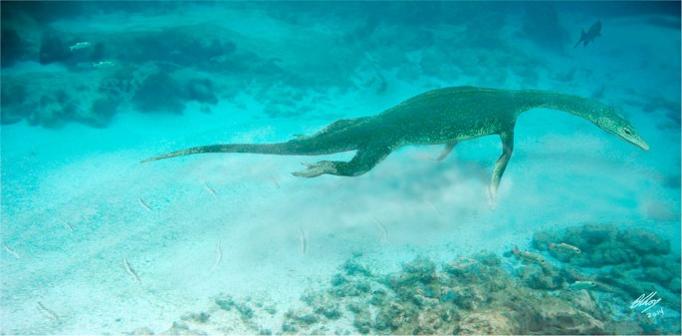Figure 8: Seabed scene, Luoping, 245 Myr ago. The nothosaur,Lariosaurus, prowls along the seafloor, searching for lobsters and fishes hiding in the soupy bottom mud. She uses her front paddles to punt along, keeping at the right height for feeding, and leaving theDikoposichnustrack behind. The reconstruction scene is based on the tracks, and our identification of the most likely track maker, as well as an interpretation of a likely function. Original artwork Brian Choo, 2014. Figure 8: Seabed scene, Luoping, 245 Myr ago. The nothosaur, Lariosaurus , prowls along the seafloor, searching for lobsters and fishes hiding in the soupy bottom mud. She uses her front paddles to punt along, keeping at the right height for feeding, and leaving the Dikoposichnus track behind. The reconstruction scene is based on the tracks, and our identification of the most likely track maker, as well as an interpretation of a likely function. Original artwork Brian Choo, 2014. Full size image The Panxian nothosaurs are Lariosaurus hongguoensis (Jiang et al . [18] ) known from a more or less complete skeleton (preserved length is 58 cm), and Nothosaurus yangjuanensis (Jiang et al . [19] ), known only from a skull (34.8 cm). The skull length of Lariosaurus hongguoensis is about 8 cm, the restored complete body length is about 80 cm, and the width of torso+outstretched paddle should be about 40 cm. In Nothosaurus yangjuanensis , the preserved skull suggests an estimated body length of 2.68 m, and the width of torso+outstretched paddle could reach 1.74 m. Larger, isolated remains of individual limb bones and vertebrae suggest that Panxian and Luoping nothosaurs could reach up to 5 m in total length and 3 m in width. With trackway widths of 35–42 cm and 50–67 cm, the smaller Luoping Dikoposichnus paddle marks could have been produced by Lariosaurus hongguoensis , and the larger prints by either species, perhaps small examples of Nothosaurus yangjuanensis . The swimming mode of Jurassic and Cretaceous plesiosaurs and pliosaurs has been studied extensively, and it has been suggested that they alternately rowed, paddled or ‘flew’ through the water, using their forelimbs to generate forward propulsion [1] , [2] , [3] , [4] , [5] . In earlier studies, several authors had assumed that nothosaurs used similar limb-dominated swimming modes, and this is confirmed in a study [20] of nothosaur bone histology in which the humerus shows morphological and bone histological features consonant with stresses associated with vigorous paddling. It is likely then that nothosaurs used their fore paddles to provide the power stroke in swimming. The most recent models and experiments in plesiosaurs [5] suggest that synchronous, or semi-synchronous, movements of right and left paddles provided the most efficient mode. This independent discovery that synchronous movements of the fore paddles is a likely swimming mode matches the finding here that most trackways show such paddle movements, although others show the asynchronous or alternate mode. Here in the footprint beds of the Middle Triassic at Luoping, we envisage nothosaurs of various sizes swimming close to the seabed, foraging along the seafloor and flushing crustaceans and fishes out of hiding, which they then snapped up ( Fig. 8 ). The needle-like teeth of the nothosaurs indicate a diet of relatively soft-bodied prey, so the bivalves, gastropods, echinoderms and brachiopods of the Luoping marine fauna [13] are presumably ruled out. Also ruled out are the belemnoids, ammonoids and conodonts, which were likely nektonic, not benthic. This leaves crustaceans and fishes, which were abundant [13] , and include many forms that presumably lurked in the seabed murk, feeding on organic matter or small prey in and above the consolidated sediment. Invertebrate burrows associated with the tracks (see above) indicate the presence of other soft-bodied animals, such as worms, that might also have been eaten by the foraging nothosaurs. This compares and contrasts with the inferences from a find of stomach contents from Lower Cretaceous elasmosaurids that includes remains of many benthic invertebrates, predominantly bivalve shell fragments, as well as remains of gastropods and pieces of crinoid [21] : this find was presented as evidence for bottom-feeding as a mode of life for some Cretaceous plesiosaurs, perhaps analogous to the feeding mode proposed here for their sauropterygian ancestors, the Triassic nothosaurs. Previous work has indicated that the surface of the seafloor at the time of the Luoping biota was covered by microbial mats [13] , [22] , which probably substantially contributed to the preservation of the trackways by binding and biostabilisation of the sediment surface [23] , [24] . We envisage that the nothosaurs positioned themselves at the right level by feeling for the surface of microbial mat, and then punted forwards at slow speeds by rowing, or alternately striding, with their forelimbs ( Figs 7 and 8 ). Such a hands-down posture kept the head clear of bottom turbulence, and the animal could dart its slender head from side to side, snatching likely prey in its jaws lined with needle-sharp teeth. The straight-line and curving trackways produced by the punting nothosaurs ( Fig. 2 ) may then reflect routes across the seafloor that seemed to yield maximum prey volumes. Marine reptile tracks of this kind have not been reported before, and indeed markings or impressions of any kind that might have been produced by any of the Mesozoic marine reptiles are very rare. The only trace fossils previously attributed to sauropterygians include foraging gutters and walking prints. The gutters, from the Late Jurassic (Callovian) of Liesberg, Switzerland, were 60-cm wide and up to 9-m long, and supposedly produced by plesiosaurs or ichthyosaurs, forcing their heads through the seabed mud (Geister [9] ). The second reported example [10] comprises prints, called Accordiichnus natans , from the Early Jurassic of the River Burano Valley, Cantiano, Italy, which are alternating and show impressions of hands and feet. The impressions of the hands are widely spaced and pear-shaped, whereas the foot impressions are crescentic and comprise five separate toe imprints, running in a tight zig-zag along the midline of the trace. They were ascribed to a plesiosaur that was walking on the seabed, placing its front paddles firmly on the seabed, and the hindlimbs strangely impressing only the toe tips, rather than a full paddle, into the mud. Arduini [25] has identified similar tracks from shallower marine limestones as undertracks of sauropodomorphs [26] , so it is not clear that Accordiichnus is a convincing marine reptile track. Much more convincing are a number of reports of trackways produced by Mesozoic marine turtles. The best example is a series of trackways made by a large swimming/paddling turtle, from the Late Jurassic of Cerin, France [27] . The trackway comprises paired fore- and hind-paddle prints, the hands making slightly transverse imprints, showing all five digits along the anterior margin, and the feet producing elongate, slightly curved, deep grooves in the substrate subparallel to the direction of travel. Like our Dikoposichnus tracks, the animal was not supporting its weight, but was using the seabed to provide purchase as it punted itself along. Unlike Dikosopichnus , the trackways generally comprise impressions of fore- and hind-paddles, and the shapes and orientations of those imprints are entirely different. A further example is a single manus imprint from the Early Cretaceous of northern Germany [28] , similar in shape to the Cerin examples, and providing evidence that it was produced by a swimming turtle, paddling itself along by digging the tips of its fingers into the seabed mud. These fossil tracks [27] , [28] are identified as those of paddling, water-supported turtles based on direct comparison with punting tracks produced by the modern leatherback turtle [29] , and they differ from the regular quadrupedal walking tracks of turtles on land [30] . Other tetrapod swimming traces include a variety of swimming, wading and walking tracks from Early Permian lacustrine deposits from Oklahoma, USA [31] . The swimming tracks include two morphologies, crescent-shaped, narrow impressions representing manus and pes prints made by an animal with webbed feet, and toe scratches parallel to the direction of locomotion, as seen also in swimming traces of some dinosaurs [32] , [33] , [34] , [35] , [36] and pterosaurs [37] . The final example is the trace fossil Mesosaurichnus from the Early Permian Irati Formation of Brazil, comprising sets of narrow grooves made by wide, sweeping kicks of the hindlegs of Mesosaurus swimming using lateral undulations of the tail [38] . It is surprising that such paddle imprints made by marine reptiles have not been widely reported before. Sinuous tracks made by fishes, on the other hand, are much better known, primarily the traces called Undichna produced by the tips of the paired fins of actinopterygians and sarcopterygians, from the Early Devonian to Pleistocene, and even recent [12] . Most records are from freshwater settings, where conditions for preservation might have been more favourable than in many marine facies. Marine examples include specimens from the Triassic of Germany and Italy. Digital mapping After excavation and thorough cleaning, the track-bearing surface was first marked out 1 m 2 and measured and highlighted with a chalk-covered string, then photographed overall. The whole area was photographed, square-by-square, using a camera mounted directly on a tripod. The surface was then scanned and mapped, using principles of laser triangulation, with a Minolta Vivid 910 non-contact 3D digitizer. Two lenses (wide-angle and telephoto) were used alternately to acquire the data of the full field and of single footprints. Then, the three-dimensional (3D) cloud data of the large- and small-field views were embedded and merged in Innovmetric PolyWorks software to capture the whole surface. The final results indicate both the distribution of the imprints and the details of each trackway in different directions, which provide high-resolution 3D digital models. Track measurement All imprints and tracks were measured in the field. Trackway widths were measured with cloth tape measures, to the nearest centimetre. Dimensions of individual imprints were measured with plastic rulers to the nearest millimetre. These imprint measurements were later checked from the scanned track model, by using measurement tools in PolyWorks. The dense and high accuracy (maximum error of 0.2 mm) 3D point data of the footprint site was digitized by Zhang et al . [39] , and Zhang and Su [40] from Sichuan University, mainly focusing on 3D metrology, with their 3D Laser scanner and professional software. Nomenclatural acts This published work and the nomenclatural acts it contains have been registered in ZooBank, the proposed online registration system for the International Code of Zoological Nomenclature (ICZN). The ZooBank LSIDs (Life Science Identifiers) can be resolved and the associated information viewed through any standard web browser by appending the LSID to the prefix ‘ http://zoobank.org/ ’ for this publication. The LSIDs for this publication is: NomenclaturalActs/D30022CA-FC6C-4FD3-BA86-2CA6D22720E8. How to cite this article: Zhang, Q. Y. et al . Nothosaur foraging tracks from the Middle Triassic of southwestern China. Nat. Commun. 5:3973 doi: 10.1038/ncomms4973 (2014).